A multi-structural and multi-functional integrated fog collection system in cactus Multiple biological structures have demonstrated fog collection abilities, such as beetle backs with bumps and spider silks with periodic spindle-knots and joints. Many Cactaceae species live in arid environments and are extremely drought-tolerant. Here we report that one of the survival systems of the cactus Opuntia microdasys lies in its efficient fog collection system. This unique system is composed of well-distributed clusters of conical spines and trichomes on the cactus stem; each spine contains three integrated parts that have different roles in the fog collection process according to their surface structural features. The gradient of the Laplace pressure, the gradient of the surface-free energy and multi-function integration endow the cactus with an efficient fog collection system. Investigations of the structure–function relationship in this system may help us to design novel materials and devices to collect water from fog with high efficiencies. Many plants and animals have evolved intriguing wetting properties; these special abilities result from the unique micro- and nano-scale structural features on their surfaces [1] , [2] , [3] , [4] , [5] , [6] . For example, certain beetles living in the Namib Desert can collect water from the fog on their backs [4] . Spider silks can also harvest water from humid air using the periodic spindle-knots and joints [5] . The gradient of surface-free energy [7] , [8] and gradient of Laplace pressure [9] , [10] , [11] are believed to be the primary driving forces behind these phenomena. Many members of the Cactaceae family can survive in highly arid deserts [12] . In addition to the adaptive characteristics that minimise water loss [13] , [14] , some species appear to use fog as an additional water supply by using spines [15] , [16] , [17] that fulfil multiple functions [14] , [15] , [18] . Despite the considerable amount of research that has been performed on the Cactaceae family, the process of fog harvesting using spines is still poorly understood. Here we demonstrate that the cactus O. microdasys , which originates from the Chihuahua Desert, has an integrated multi-functional system that facilitates efficient fog collection. This unique fog collection system can be attributed to the integration of its multi-level surface structures. Appearance and surface structures The optical images of a representative O. microdasys stem in Fig. 1a–c illustrate the structural characteristics of this plant. Clusters of needle-like spines and trichomes grow as a well-distributed array on the stem’s surface with distances ranging from ∼ 7 to 23 mm ( Fig. 1a ). Together, the top-view image in Fig. 1b and the side-view image in Fig. 1c illustrate a single cluster containing ∼ 100 spines. These spines grow in arbitrary directions with an average angle of 18.1±5.3° between the nearest two spines, forming a hemispherical structure. The spines range from ∼ 800 to 2,500 μm in length and ∼ 30 to 65 μm in diameter in the middle portion. The dotted line in Fig. 1c shows the trichomes at the base of the spines; these trichomes also form a hemispherical structure (see also Supplementary Fig. S1 ). To investigate these structures in detail, we used a scanning electron microscope (SEM) to observe an individual spine (see Fig. 1d–h , Supplementary Fig. S2 , and Supplementary Fig. S3 ). 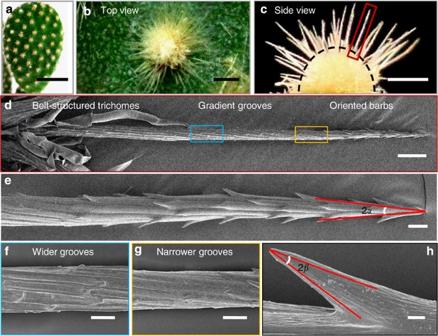Figure 1: Appearance and surface structures of the cactus. (a) Optical image of a plant ofO. microdasysstem covered with well-distributed clusters of spines and trichomes. (b,c) Magnified optical images of a single cluster with spines growing from the trichomes in the top (b) and side (c) view. (d) SEM image of a single spine divided into three regions, the tip (e) with an apex angle (2α) and oriented barbs, the middle (f,g) with gradient grooves, and the base with belt-structured trichomes. (f,g) Magnified images of regions near the base and tip of the cactus spine, respectively. The microgrooves near the base are wider and sparser than those near the tip. (h) Magnified image of a single barb with an apex angle (2β) covering the tip of the spine (e). Scale bars, 5 cm (a), 500 μm (b,c), 100 μm (d), 20 μm (e–g) and 2 μm (h). Figure 1d shows that the spine is composed of three parts with different structural features, the tip contains oriented barbs, the middle contains gradient grooves and the base contains belt-structured trichomes. The spine has a conical shape with an apex angle (2 α ) of 12.3±1.6° ( Fig. 1e ). The magnified image of the barb in Fig. 1h also reveals a conical shape (apex angle 2 β : 19.5±3.3°) with aligned grooves. The magnified images of the middle portion of the spine reveal multi-level grooves. The first-level grooves (the epidermal cells of the cactus spines) [19] , [20] are microgrooves and have a gradient in width along the spine, from an average of ∼ 6.8 μm near the base to an average of ∼ 4.3 μm near the tip ( Fig. 1f–g and Supplementary Fig. S2a,b ). The second-level grooves (the folding sculptures of the epidermal cell) [19] are primarily submicrogrooves lacking an obvious gradient in width and are characterized with a constant value of ∼ 0.6 μm over the entire length of the spine ( Supplementary Fig. S3 ). The subtle integration of these structures (that is, conical spines and barbs, oriented barbs, gradient grooves and belt-structured trichomes) may contribute to the superior ability of these structures to collect fog. Figure 1: Appearance and surface structures of the cactus. ( a ) Optical image of a plant of O. microdasys stem covered with well-distributed clusters of spines and trichomes. ( b , c ) Magnified optical images of a single cluster with spines growing from the trichomes in the top ( b ) and side ( c ) view. ( d ) SEM image of a single spine divided into three regions, the tip ( e ) with an apex angle (2 α ) and oriented barbs, the middle ( f , g ) with gradient grooves, and the base with belt-structured trichomes. ( f , g ) Magnified images of regions near the base and tip of the cactus spine, respectively. The microgrooves near the base are wider and sparser than those near the tip. ( h ) Magnified image of a single barb with an apex angle (2 β ) covering the tip of the spine ( e ). Scale bars, 5 cm ( a ), 500 μm ( b , c ), 100 μm ( d ), 20 μm ( e – g ) and 2 μm ( h ). Full size image Fog collection ability The fog collection ability of the cactus O. microdasys was investigated using a saturated fog flow with a velocity of ∼ 20 to 30 cm s −1 (see Methods); the movement of the water drops was recorded by a charge-coupled device camera in time-lapse mode [5] . We placed a single spine at multiple tilt angles (90°, 45°, −45°, −90° and 0°) to determine the effects of the spine’s growing direction on the directional movement behaviour of the water drops ( Fig. 2 ). For each case, even when the spine was vertically fixed with the tip pointing down ( Fig. 2d ), the water drops were directionally driven from the tip to the base side of the spine (black arrows in Fig. 2 and Supplementary Movie 1 ). These results indicate that the gravitational force of the water drop has little effect on the directional water collection performance. The spines’ directions of growth from the cactus stem were not apparently a key factor in the directional movement of the water drops. 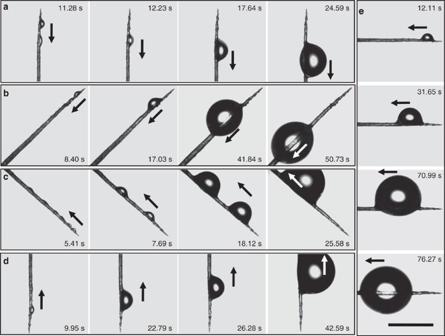Figure 2:In situoptical microscopic observation of the directional water collection on the cactus spine placed at various angles. (a–e) A spine placed in fog with the following tilt angles: 90°, 45°, −45°, −90° and 0°, respectively. The deposited water drops were driven from the tip to the base of the spine, even with the spine vertically fixed with the tip pointing down (d). Scale bar, 500 μm. Figure 2: In situ optical microscopic observation of the directional water collection on the cactus spine placed at various angles. ( a – e ) A spine placed in fog with the following tilt angles: 90°, 45°, −45°, −90° and 0°, respectively. The deposited water drops were driven from the tip to the base of the spine, even with the spine vertically fixed with the tip pointing down ( d ). Scale bar, 500 μm. Full size image Water collection process To determine the function of the barbs, spines and trichomes in the water collection process, we utilized a horizontal spine for our investigations ( Fig. 3 ). By focusing on the behaviour of the water drops on the tip side of a spine covered with several oriented barbs, we observed the initial, simultaneous deposition of tiny water drops on the barbs (drop 1) and the spine (drop 2) (see Fig. 3a ). As the deposition proceeded, growing drop 1 moved towards the base of the barb and coalesced with drop 2, forming the larger drop 1+2 (arrows in Fig. 3a ). With a continuous deposition, drop 1+2 further coalesced with drop 3, which had been deposited on the adjacent barb. After water drop 1 moved away from the barb, a new cycle of water deposition and directional collection began. This process can be seen in Fig. 3a , with additional water drop 1′ depositing in the same location as the original drop 1. During this process, the gradient of the Laplace pressure between the two sides causes the water drops on the barbs to continuously move towards the base of the barbs. 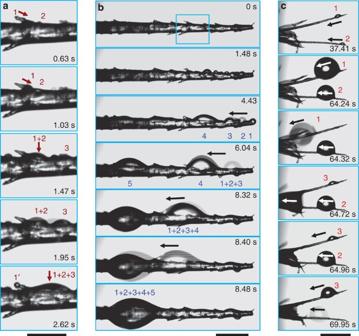Figure 3:In situoptical microscopic observation of the detailed water collection process on a single horizontal spine and two adjacent spines with trichomes. (a) Continuous deposition of the water drops on the barbs and the spine. Initially, tiny water drops 1 and 2 were deposited concomitantly on the barb and the spine, respectively. Drop 1 moved toward the base of the barb with the volume increasing and coalesced with drop 2, forming larger drop 1+2. As the deposition proceeded, drop 1+2 further coalesced with drop 3 on the adjacent barb. A new cycle started when a subsequent small water drop 1′ deposited at the same location of initial drop 1. (b) Directional collection of the water drops on the spine. The deposited drop (1) and the coalesced drops (2–4) combine, moving directionally along the spine (black arrows) to form a large drop (1+2+3+4+5). (c) The behaviour of the water drops on the two adjacent spines containing trichomes. Drops 1 and 2 moved along the spines towards the base side, increasing in size. Upon contact with the trichomes at the base, the drops were absorbed immediately through the trichomes within a half second (from 64.32 to 64.72 s). After the absorption of the coalesced drops, a new cycle of water collection can begin, as observed with the tiny drop 3 at the middle of the spine. Scale bars, 50 μm (a), 100 μm (b) and 500 μm (c). Figure 3: In situ optical microscopic observation of the detailed water collection process on a single horizontal spine and two adjacent spines with trichomes. ( a ) Continuous deposition of the water drops on the barbs and the spine. Initially, tiny water drops 1 and 2 were deposited concomitantly on the barb and the spine, respectively. Drop 1 moved toward the base of the barb with the volume increasing and coalesced with drop 2, forming larger drop 1+2. As the deposition proceeded, drop 1+2 further coalesced with drop 3 on the adjacent barb. A new cycle started when a subsequent small water drop 1′ deposited at the same location of initial drop 1. ( b ) Directional collection of the water drops on the spine. The deposited drop (1) and the coalesced drops (2–4) combine, moving directionally along the spine (black arrows) to form a large drop (1+2+3+4+5). ( c ) The behaviour of the water drops on the two adjacent spines containing trichomes. Drops 1 and 2 moved along the spines towards the base side, increasing in size. Upon contact with the trichomes at the base, the drops were absorbed immediately through the trichomes within a half second (from 64.32 to 64.72 s). After the absorption of the coalesced drops, a new cycle of water collection can begin, as observed with the tiny drop 3 at the middle of the spine. Scale bars, 50 μm ( a ), 100 μm ( b ) and 500 μm ( c ). Full size image After the initial stage, the drops that were collected from the barbs or deposited directly from the fog could be observed on the tip side of the spine (identified by numbers 1–5 in Fig. 3b ). As the water deposition continued, the drops increased in size; the tip-side drops coalesced and moved directionally along the spine (black arrows in Fig. 3b ). For example, drops 1 to 2, 1+2 to 3, 1+2+3 to 4, ultimately forming a large drop 1+2+3+4+5 (see Supplementary Movie 2 ). These observations demonstrated that the water drops could move from the tip to the base of the spine with the driving forces attributed to the gradient of the surface-free energy and the gradient of the Laplace pressure. In addition, the oriented barbs on the tip side engendered an asymmetrical surface structure, similar to the butterfly wings [2] , which enabled the unidirectional rolling and spreading of the water drops [21] , [22] , further aiding the directional movement of the water drops towards the base of the spine. Figure 3c shows this directional movement in detail (see also Supplementary Figs S4 and S5 and Supplementary Movie 3 ). The individual drops that were collected on adjacent spines both moved to the base side that was covered with trichomes. The trichomes and the spines formed conical internal surfaces, similar to shorebird’s beaks [23] , which can generate a strong capillary force. When the water drops contacted the trichomes, the drops were rapidly absorbed ( Fig. 3c ). Compared with the time-consuming transportation process ( ∼ 27 s), the absorption process was rapid (within a half second). The drops on adjacent spines also coalesced into one large drop that was absorbed by the trichomes ( Supplementary Fig. S5 ). Another cycle of water collection began as drop 3 appeared on the upper spine and moved towards the trichomes. The rapid absorption process (that is, the rapid departure of the water drops) guaranteed the rapid regeneration of the fog collection process. As described in previous studies on various species, water drops can be absorbed into the stem [14] , [16] , [18] , [19] , especially in foggy areas; from there, they can be reserved in the mucilage cells containing polysaccharides with a high affinity to water that can reduce the evaporative loss [13] . The integration of the multiple functions within the spines and the trichomes, including water deposition, collection, transportation and absorption in the cactus, facilitated an efficient fog collection system. The unique structural features of the cactus, such as the spines and the barbs with aligned gradient grooves and the cooperation between the spines and the trichomes, contributed to this system’s excellent functioning. To characterize the structure–function relationship in this efficient fog collection process, we propose a potential mechanism. 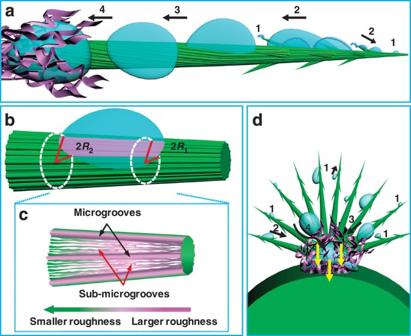Figure 4: Mechanism of the fog collection on the cactus. (a) An overview of the efficient fog collection system ofO. microdasysprogressing from ‘1 Deposition’ on the barbs and the spine to ‘2 Collection’ on the tip of the spine, ‘3 Transportation’ on the gradient grooves, and ‘4 Absorption’ upon contact with the trichomes. (b,c) Analysis of the driving forces arising from the gradient of the Laplace pressure and the gradient of the surface-free energy. A water drop on a conical spine should move towards the base side with the larger radius (R2) due to the relatively smaller Laplace pressure (b). In addition to the conical shape, the surface of the spine was covered with multi-level grooves. The gradient of the microgrooves was sparser near the base than near the tip of the spine (as indicated by the black arrows). The aligned submicrogrooves were similar along the spine as indicated by the red arrows (c). This gradient of the microgrooves produced a gradient of roughness, contributing to a gradient of the surface-free energy along the spine, driving the water drops towards the base side. (d) Cooperation among the multiple spines, the multiple trichomes and the spines-trichomes. The water drops that progress through the ‘1 Deposition’, ‘2 Collection’ and ‘3 Transportation’ processes are quickly absorbed into the cactus stem upon contact with the trichomes (‘4 Absorption’). Figure 4a shows an overview of the entire process of fog collection. ‘Deposition’ initially occurs on the barb and the spine, with the water drops moving directionally along them. As the deposition proceeds and the water drops coalesce, these drops increase in size, leaving from the tip side of the spine (‘Collection’). The bigger drops are then further transported along the gradient grooves (‘Transportation’) and absorbed through the trichomes at the base of the spines (‘Absorption’). The gradient of the Laplace pressure arising from the conical shape of the spine and the gradient of the surface-free energy arising from the gradient of the surface roughness along the spine are the two forces that drive the directional movement of the water drops. Figure 4: Mechanism of the fog collection on the cactus. ( a ) An overview of the efficient fog collection system of O. microdasys progressing from ‘1 Deposition’ on the barbs and the spine to ‘2 Collection’ on the tip of the spine, ‘3 Transportation’ on the gradient grooves, and ‘4 Absorption’ upon contact with the trichomes. ( b , c ) Analysis of the driving forces arising from the gradient of the Laplace pressure and the gradient of the surface-free energy. A water drop on a conical spine should move towards the base side with the larger radius ( R 2 ) due to the relatively smaller Laplace pressure ( b ). In addition to the conical shape, the surface of the spine was covered with multi-level grooves. The gradient of the microgrooves was sparser near the base than near the tip of the spine (as indicated by the black arrows). The aligned submicrogrooves were similar along the spine as indicated by the red arrows ( c ). This gradient of the microgrooves produced a gradient of roughness, contributing to a gradient of the surface-free energy along the spine, driving the water drops towards the base side. ( d ) Cooperation among the multiple spines, the multiple trichomes and the spines-trichomes. The water drops that progress through the ‘1 Deposition’, ‘2 Collection’ and ‘3 Transportation’ processes are quickly absorbed into the cactus stem upon contact with the trichomes (‘4 Absorption’). Full size image A water drop can be driven by chemical [7] , [8] , thermal [24] , [25] and shape [9] , [26] gradients. Specifically, a drop on a conical-shaped surface is often driven to the side with the larger radius due to the gradient of the Laplace pressure [9] . As illustrated in Fig. 4b , a cactus spine can be considered as a conical object with aligned grooves. This type of conical shape generates a Laplace pressure difference (Δ P curvature ) between the two opposite sides of the drop [5] , [9] as follows: where R is the local radius of the spine ( R 1 and R 2 are the local radii of the spine at the two opposite sides of the drop), γ is the surface tension of water, R 0 is the drop radius, α is the half-apex angle of the conical spine, and d z is the incremental radius of the spine ( Fig. 4b ). The Laplace pressure on the region near the spine’s tip (small radius R 1 ) is larger than that near the base (large radius R 2 ). This difference (Δ P curvature ) within the water drop initiates a driving force that makes the drop move from the tip to the base side along the cactus spine. In addition to the gradient of the Laplace pressure, the gradient of the surface-free energy is another driving force. Specifically, the microgrooves on the cactus spines have a gradient in width. The microgrooves are sparser near the base (less rough) than near the tip (rougher) of the spine ( Fig. 4c and Supplementary Fig. S2 ). This roughness can be described using Wenzel’s equation [27] as follows: where r is the roughness factor defined as the ratio of the actual surface area to the geometric projected area of a rough surface, and θ and θ w are the intrinsic and apparent contact angles, respectively. The gradient of roughness generates a gradient of wettability, (that is, a gradient of surface-free energy) [28] , [29] , [30] . For the surface of the cactus spines covered with vegetable wax [19] , the tip is rougher and more hydrophobic; whereas the base is less rough and less hydrophobic (see Supplementary Fig. S6 ). In other words, the tip of the spine has a lower surface-free energy than the base. This gradient of the surface-free energy produces a driving force F , driving the water drops collected on the tip directionally towards the base [5] as described as follows: where θ A and θ R are the advancing and receding contact angles of water drops on the middle of the spine, respectively, and d l is the integral variable along the length of the middle of the spine from the region near the tip ( l tip ) to the region near the base ( l base ). The roughness arising from the microgrooves on the cactus spine enhances the gradient of the Laplace pressure (see Supplementary Fig. S7 ), contributing to the movement of the water drops along the cactus spines. The aligned grooves can also generate an anisotropic contact angle hysteresis (CAH) [31] , [32] in the direction parallel or perpendicular to the grooves, enhancing the directional movement of the water drops along the grooves on the barbs and spines (See Supplementary Fig. S8 ). Specifically, a water drop moves more readily in the direction that is parallel to the aligned structures than in other directions [33] . The drop has a continuous, three-phase contact line along the grooves that reduces the energy barrier and therefore facilitates the spreading and moving of the drop [34] . Without a gradient in width along the cactus spine, the submicrogrooves further enhance this anisotropic CAH ( Supplementary Fig. S3 ), facilitating the directional movement of the water drops along the barbs and the spines. In addition to the aligned grooves, the oriented barbs reduce the drop’s ability to spread or move towards the tip side with the barbs, facilitating movement towards the base side lacking barbs. With an anisotropic CAH [35] , a water drop on a surface with asymmetrical structures has a preferred direction to spread or move [2] , [21] , [22] . Because the barbs orient in the direction towards the spine’s base ( Fig. 1e ), the water drops prefer to spread and move along the oriented direction of the barbs. This CAH difference further aids the growth and movement of the water drops to the base side of the spine under deposition. These fog collection abilities have been examined using the mechanisms of a single spine. To extend this approach to a more complete system with tens of spines and trichomes in a single cluster ( Fig. 1b ), the cooperation among spines-trichomes, multiple spines and multiple trichomes in the collection process ( Fig. 4d ) must also be considered. In addition, the array of multiple clusters on the stem surface ( Fig. 1a ) may further enhance the fog collection ability. The integration of the multi-level structures and the consequent integration of the multi-functional abilities, including the deposition, collection, transportation and absorption of the water drops, may provide O. microdasys with an efficient fog collection system. The investigation into the structure–function relationship within this system may offer systematic opinions that can be used to design novel materials and devices to efficiently collect fog. By mimicking the primary characters of the areole system of O. microdasys and considering the existing artificial fog collectors [36] , [37] , [38] , an artificial system with similar mechanisms to cactus is currently being developed, as shown in Supplementary Fig. S9 and Supplementary Note 1 . Owing to its high efficiency and portability, this artificial system may find applications in the self water supply for plants and human beings that live in arid areas ( Supplementary Fig. S9 ). Materials The cactus ( Opuntia microdasys ) was purchased from the Chinese Academy of Agricultural Sciences, Beijing, China. The clusters of the spines and trichomes, and the single spine were carefully selected and fixed on the sample frame. Characterization of the microstructures The optical images of the cactus were recorded by a digital camera (Canon Powershot A1100IS). The microstructures of the spines, the barbs and the trichomes were observed by a field-emission scanning electron microscope (JEOL, JSM-6700 F, Japan) at an accelerating voltage of ∼ 3.0 KV. Fog collection experiment and observation The cactus spine was carefully fixed on a frame and investigated under a saturated fog flow with a velocity of ∼ 20–30 cm s −1 (by an ultrasonic humidifier using Milli-Q water). The behaviour of the water drops was recorded by the optical contact angle meter system with charge-coupled device components. (OCA 40, Dataphysics Instruments GmbH, Germany). How to cite this article: Ju, J. et al. A multi-structural and multi-functional integrated fog collection system in cactus. Nat. Commun. 3:1247 doi: 10.1038/ncomms2253 (2012).